TRPV4 channel activity is modulated by direct interaction of the ankyrin domain to PI(4,5)P2 Mutations in the ankyrin repeat domain (ARD) of TRPV4 are responsible for several channelopathies, including Charcot–Marie–Tooth disease type 2C and congenital distal and scapuloperoneal spinal muscular atrophy. However, the molecular pathogenesis mediated by these mutations remains elusive, mainly due to limited understanding of the TRPV4 ARD function. Here we show that phosphoinositide binding to the TRPV4 ARD leads to suppression of the channel activity. Among the phosphoinositides, phosphatidylinositol-4,5-bisphosphate (PI(4,5)P 2 ) most potently binds to the TRPV4 ARD. The crystal structure of the TRPV4 ARD in complex with inositol-1,4,5-trisphosphate, the head-group of PI(4,5)P 2 , and the molecular-dynamics simulations revealed the PI(4,5)P 2 -binding amino-acid residues. The TRPV4 channel activities were increased by titration or hydrolysis of membrane PI(4,5)P 2 . Notably, disease-associated TRPV4 mutations that cause a gain-of-function phenotype abolished PI(4,5)P 2 binding and PI(4,5)P 2 sensitivity. These findings identify TRPV4 ARD as a lipid-binding domain in which interactions with PI(4,5)P 2 normalize the channel activity in TRPV4. The nonselective cation channel TRPV4 is a member of the vanilloid subfamily of the transient receptor potential (TRP) channels. TRPV4 has multiple regulatory sites and modes of activation, enabling it to respond to various stimuli. TRPV4 is activated by physical stimuli, including moderate heat, cell swelling and shear stress, by endogenous chemicals, such as anandamide, arachidonic acid (AA) and its cytochrome P450-derived metabolites (epoxyeicosatrienoic acids, EETs), and by numerous exogenous chemical ligands, such as 4α-phorbol-12,13-didecanoate (4α-PDD) [1] , [2] . The sensitivity of TRPV4 to cell swelling and shear stress is mediated by the activation of phospholipase A 2 (PLA 2 ) and the subsequent production of AA and EETs [2] , [3] . Recent studies using Trpv4 knockout mice have suggested the functional importance of TRPV4 in the central nervous system, nociception and bone formation [1] . The amino (N)- and carboxy (C)-terminal cytoplasmic regions of TPRV4 contain a variety of functional domains [1] . For example, the N-terminus of TRPV4 features a characteristic ankyrin repeat domain (ARD), consisting of six ankyrin repeats. The proline-rich region just upstream of the first ankyrin repeat interacts with PACSIN3, which associates with cytoskeletal proteins [4] . The TRPV4 C-terminal tail contains additional functional domains, such as a TRP box, a calmodulin-binding site and a binding site for cytoskeletal proteins. At present, no crystallographic or nuclear magnetic resonance data are available that can shed light on the atomic structure of functional TRPV4. However, the structure of rat TRPV4 was analyzed at 3.5 nm resolution by cryo-electron microscopy [4] , and the ARD appeared to lie on the membrane in an oblique orientation. Mutations in TRPV4 are associated with a wide spectrum of inherited diseases. Recent reports have identified TRPV4 mutations as the direct cause of primarily autosomal dominant neuropathies and skeletal dysplasias, such as congenital distal spinal muscle atrophy (CDSMA), scapuloperoneal spinal muscular atrophy (SPSMA) and Charcot–Marie–Tooth disease (CMT) type 2C (CMT2C) [1] , [2] . CMT is the most common inherited neuromuscular disorder, affecting at least 1 in 2,500 people, and is a genetically heterogeneous disorder with common clinical phenotypes, such as distal muscle weakness and atrophy, sensory loss and foot deformities [5] , [6] . The mutations in TRPV4 are the most recently identified CMT subtype, in terms of genetic locus [1] , [2] . Previous studies have suggested that the gain-of-function mutations of TRPV4 in these diseases, which exhibit increased basal and maximum Ca 2+ channel activities, are clustered within the TRPV4 ARD and affect arginine residues, especially at the R232C, R269C/H, R315W, R316C/H positions [7] , [8] , [9] , [10] . The increased Ca 2+ influx and subsequent Ca 2+ overload associated with these mutations are thought to be the cause of cell death, and have been proposed as a mechanism for peripheral axonal degeneration in TRPV4-dependent neuropathies [9] , [10] . However, the molecular mechanism underlying the increased activity of these mutants has remained unknown. Therefore, elucidation of the TRPV4 ARD regulation at the molecular level is essential for understanding the mechanisms for diseases associated with TRPV4 mutations. Over the last two decades, the molecular basis for CMT has become clearer, with the identification of more than 30 causative genes [11] . Recent research into the genetic basis and the molecular disease mechanisms of CMT has highlighted phosphoinositides as key regulatory molecules in a variety of CMT subtypes [12] . Phosphoinositides are essential components of membrane lipids and regulate fundamental biological processes, including cell growth, membrane trafficking and cytoskeletal dynamics, through binding to effector proteins [13] , [14] , [15] . Phosphoinositides also act as precursors of second messengers, such as inositol-1,4,5-trisphosphate (IP 3 ) and diacylglycerol (DAG), which are both produced through the hydrolysis of phosphatidylinositol-4,5-bisphosphate (PI(4,5)P 2 ) by phospholipase C (PLC) isoforms [16] . There are phosphoinositide-binding domains in several proteins linked to CMT, including dynamin2 (ref. 17 ), KIF1Bβ [18] , neurofilament (NEFL) [19] , Pleckstrin homology (PH) domain containing, family G member 5 (PLEKHG5) [20] and Frabin/FGD [21] , [22] . Notably, mutations in the PI(4,5)P 2 -binding domains of dynamin2 (ref. 17 ) and PLEKHG5 (ref. 20 ) have been identified as the causes of CMT. In addition, several different CMT subtypes occur due to mutations in phosphoinositide-specific phosphatases [12] , including MTMR2, MTMR13 and FIG4. Thus, increasing evidence supports the close relationships of CMT-causative proteins with phosphoinositide signalling. It is possible that phosphoinositides are involved in CMT2C. The CMT2C mutations of TRPV4 are mainly located in the ARD. Although the ARD is generally responsible for protein–protein interactions, these studies connecting the relationships between CMT2C and phosphoinositides prompted us to examine the interaction of the TRPV4 ARD with phosphoinositides. In this study, we show that the ARD of TRPV4 most potently binds to PI(4,5)P 2 . Our structural analyses and functional assays suggest that the TRPV4 ARD interacts with the inositol head group of PI(4,5)P 2 , which negatively regulates the TRPV4 channel activity. Notably, the majority of the disease-associated mutants that exhibit a gain-of-function phenotype show decreased binding and sensitivity to PI(4,5)P 2 , providing a correlation between the PI(4,5)P 2 sensitivity and the disease phenotypes. Membrane lipid-binding ability of TRPV ARDs We examined the ability of the TRPV4 ARD to bind to a series of membrane lipids, including phosphoinositides. The ARD of TRPV4 bound to phosphoinositides, and a relatively strong affinity to PI(4,5)P 2 was revealed by the liposome co-sedimentation assay ( Fig. 1a ). The TRPV1 ARD bound to lipids; however, the specific binding of the TRPV1 ARD to particular lipids was not observed ( Fig. 1a ). 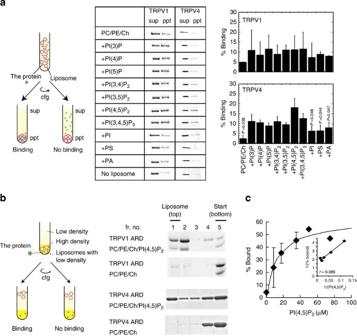Figure 1: Membrane lipids that bind to the TRPV4 ARD. (a) Liposome co-sedimentation assay. The ARDs of TRPV1 and TRPV4 were prepared, and their lipid binding was examined. The presence of protein in the pellet (ppt) indicated protein binding. Control experiments without liposomes were also performed. The bound proteins are shown as mean±s.e.m. (n=5).Pvalues relative to PI(4,5)P2are shown. PA, phosphatidic acid; PC, phosphatidylcholine; PE, phosphatidylethanolamine; PI, phosphatidylinositol; PI(3)P, phosphatidylinositol 3-phosphate; PI(4)P, phosphatidylinositol 4-phosphate; PI(5)P, phosphatidylinositol 5-phosphate; PI(3,4)P2, phosphatidylinositol 3,4-bisphosphate; PI(3,5)P2, phosphatidylinositol 3,5-bisphosphate; PI(4,5)P2, phosphatidylinositol 4,5-bisphosphate; PI(3,4,5)P3, phosphatidylinositol 3,4,5-trisphosphate; PS, phosphatidylserine. PI-phosphate, PI- bisphosphate, and PI- trisphosphate were included in 5.5, 5 or 4.5 mol% or 9 weight%. (b) Liposome floating assay. The binding of TRPV1 and TRPV4 to PI(4,5)P2-containing liposomes was examined. All fractions were examined, and the appearance of protein in the top fraction indicates the protein–lipid interaction. (c) Determination of the dissociation constant. The bound liposome in the floating assay was plotted against the amount of PI(4,5)P2. 1/[% bound TRPV4 ARD] and 1/[PI(4,5)P2] are also plotted, with their correlation coefficients (r). The amount of PI(4,5)P2in total lipids was increased in this assay from 0 to 15% (75 μM, one-half of the total PI(4,5)P2, because of the lipid bilayer). The dissociation constant was determined from the intercept and the slope of 1/[% bound TRPV4 ARD] and 1/[PI(4,5)P2] (n=3, 2, 4, 1 and 2 for 8.75, 17.5, 35, 50 and 75 μM PI(4,5)P2, respectively). Data points are mean±s.e.m. Figure 1: Membrane lipids that bind to the TRPV4 ARD. ( a ) Liposome co-sedimentation assay. The ARDs of TRPV1 and TRPV4 were prepared, and their lipid binding was examined. The presence of protein in the pellet (ppt) indicated protein binding. Control experiments without liposomes were also performed. The bound proteins are shown as mean±s.e.m. ( n =5). P values relative to PI(4,5)P 2 are shown. PA, phosphatidic acid; PC, phosphatidylcholine; PE, phosphatidylethanolamine; PI, phosphatidylinositol; PI(3)P, phosphatidylinositol 3-phosphate; PI(4)P, phosphatidylinositol 4-phosphate; PI(5)P, phosphatidylinositol 5-phosphate; PI(3,4)P 2 , phosphatidylinositol 3,4-bisphosphate; PI(3,5)P 2 , phosphatidylinositol 3,5-bisphosphate; PI(4,5)P 2 , phosphatidylinositol 4,5-bisphosphate; PI(3,4,5)P 3 , phosphatidylinositol 3,4,5-trisphosphate; PS, phosphatidylserine. PI-phosphate, PI- bisphosphate, and PI- trisphosphate were included in 5.5, 5 or 4.5 mol% or 9 weight%. ( b ) Liposome floating assay. The binding of TRPV1 and TRPV4 to PI(4,5)P 2 -containing liposomes was examined. All fractions were examined, and the appearance of protein in the top fraction indicates the protein–lipid interaction. ( c ) Determination of the dissociation constant. The bound liposome in the floating assay was plotted against the amount of PI(4,5)P 2 . 1/[% bound TRPV4 ARD] and 1/[PI(4,5)P 2 ] are also plotted, with their correlation coefficients ( r ). The amount of PI(4,5)P 2 in total lipids was increased in this assay from 0 to 15% (75 μM, one-half of the total PI(4,5)P 2 , because of the lipid bilayer). The dissociation constant was determined from the intercept and the slope of 1/[% bound TRPV4 ARD] and 1/[PI(4,5)P 2 ] ( n =3, 2, 4, 1 and 2 for 8.75, 17.5, 35, 50 and 75 μM PI(4,5)P 2 , respectively). Data points are mean±s.e.m. Full size image The liposome binding to the TRPV proteins was further confirmed by a co-floating assay, in which the liposome-containing low-density media float up after centrifugation. Thus, the co-floating assay can be used to examine unstable proteins, which are precipitated by centrifugation after their aggregation. The coexistence of a protein with the floated liposomes indicates the liposome–protein interaction. The binding of the TRPV1 and TRPV4 ARDs to lipids in the membrane was confirmed, using liposomes containing PI(4,5)P 2 ( Fig. 1b ). The dissociation constant for TRPV4 and PI(4,5)P 2 was determined to be 14 μM ( r =0.985) by the liposome floating assay ( Fig. 1c ), and 43 μM ( r =0.995) by a Surface Plasmon Resonance (SPR) analysis ( Supplementary Fig. 1 ). These two values are considered to be in the range of variation because of the differences in the methods. Crystal structure of the ARD·IP 3 complex To identify the PI(4,5)P 2 -binding site, we prepared crystals of the chicken TRPV4 ARD and exposed them to a solution containing IP 3 , the head-group of PI(4,5)P 2 . The crystal structure of the chicken TRPV4 ARD (residues 133–382, corresponding to human residues 147–396) in complex with IP 3 was determined at 1.9 Å resolution by the molecular replacement method, using the reported chicken TRPV4 ARD structure (PDB ID: 3JXI [9] ) as the search model ( Fig. 2a–c , Supplementary Fig. 2 and Table 1 ). The chicken ARD structure without IP 3 was also determined at 2.0 Å resolution, for comparison. 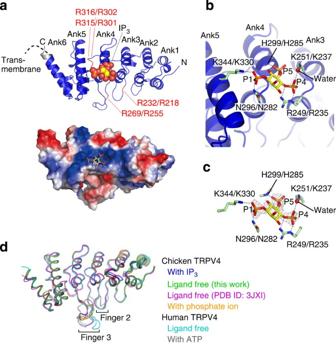Figure 2: Crystal structure of the TRPV4 ARD·IP3complex. (a) Crystal structure of the chicken TRPV4 ARD·IP3complex. IP3is shown as a sphere model. The artificially introduced regions, the N-terminal initiating Met and the C-terminal Ala3linker followed by the His6tag are coloured grey. Mutated residues identified in the inherited diseases are coloured red. The lower panel shows the surface electrostatic potentials, where red and blue represent acidic and basic characteristics, respectively. (b) The IP3-binding site. The amino-acid residues are labelled with the human/chicken numbering. Putative hydrogen bonds are shown as dashed lines. (c) The omitFO−FCmap (3.0 sigma level) of IP3is shown in a grey mesh. (d) The superimposed tube diagrams of the present and reported crystal structures of TRPV4 ARD. Chicken ARD in complex with IP3, ARD without ligand (this work), without ligand (PDB ID: 3JXI9) and in complex with phosphate ion (PDB ID: 3JXJ9) are coloured blue, green, magenta and orange, respectively. For comparison, the human ARD without ligand (PDB ID: 4DX1 (ref.23) and in complex with ATP (PDB ID: 4DX2 (ref.23) are coloured cyan and grey, respectively. The chain A molecule from each crystal structure is represented. Figure 2: Crystal structure of the TRPV4 ARD·IP 3 complex. ( a ) Crystal structure of the chicken TRPV4 ARD·IP 3 complex. IP 3 is shown as a sphere model. The artificially introduced regions, the N-terminal initiating Met and the C-terminal Ala 3 linker followed by the His 6 tag are coloured grey. Mutated residues identified in the inherited diseases are coloured red. The lower panel shows the surface electrostatic potentials, where red and blue represent acidic and basic characteristics, respectively. ( b ) The IP 3 -binding site. The amino-acid residues are labelled with the human/chicken numbering. Putative hydrogen bonds are shown as dashed lines. ( c ) The omit F O − F C map (3.0 sigma level) of IP 3 is shown in a grey mesh. ( d ) The superimposed tube diagrams of the present and reported crystal structures of TRPV4 ARD. Chicken ARD in complex with IP 3 , ARD without ligand (this work), without ligand (PDB ID: 3JXI [9] ) and in complex with phosphate ion (PDB ID: 3JXJ [9] ) are coloured blue, green, magenta and orange, respectively. For comparison, the human ARD without ligand (PDB ID: 4DX1 (ref. 23 ) and in complex with ATP (PDB ID: 4DX2 (ref. 23 ) are coloured cyan and grey, respectively. The chain A molecule from each crystal structure is represented. Full size image Table 1 Data collection and refinement statistics. Full size table The TRPV4 ARD consists of six ankyrin repeats (Ank1–6; Fig. 2a and Supplementary Fig. 3 ). The protein structure of the ARD·IP 3 complex is nearly identical to the present and reported chicken TRPV4 ARD structures without a ligand [9] ( Fig. 2d ), indicating that IP 3 binding does not affect the overall structure of ARD. On the other hand, the finger 3 conformation differs from those of the chicken TRPV4 ARD in complex with phosphate ion and the human TRPV4 ARD without a ligand [9] , [23] ( Fig. 2d ). The conformational change in finger 2 is observed upon ATP binding to the human TRPV4 ARD [9] ( Fig. 2d ). The IP 3 is located beside the Ank4 repeat and interacts with the residues from Ank3–5 via its phosphate groups (P1, P4 and P5; Fig. 2b,c ). P1 interacts with the side chains of N296/N282 (human/chicken residue numbers, respectively) in Ank4 and K344/K330 in Ank5, whereas P4 and P5 interact with the R249/R235 side chains in Ank3 and the H299/H285 main chain NH in Ank4, respectively. Furthermore, P4 forms a water-mediated interaction with the K251/K237 side chain in Ank3. We also explored the differences between the TRPV4 ARD and the TRPV1 ARD (PDB ID: 2NYJ [24] ). The surface of the TRPV1 ARD is positively charged, but the positive charges are not clustered, as compared with those in the TRPV4 ARD ( Supplementary Fig. 4 ), which might explain the lower lipid-binding selectivity of TRPV1 ( Fig. 1a ). Docking simulations of the ARD To further investigate the interaction between the TRPV4 ARD and the membrane, we tested various phosphorylated inositols, the heads of phosphoinositides, for ARD binding in silico ( Fig. 3a ). Randomly placed inositols were assessed for the binding. The candidate-binding site can be estimated by two calculated values, the cluster size and the binding energy. The size of the cluster indicates the population of inositols bound to that site. Although accurate estimation of the binding free energy for highly charged residues is challenging, the binding energy is expected to correlate with the dissociation constant, where lower energy indicates stronger binding. Notably, myo-inositol 1,4,5-trisphosphate (IP 3 ), the head of PI(4,5)P 2 , and myo-inositol 1,3,4,5-tetraphosphate, the head of PI(3,4,5)P 3 , exhibited relatively lower binding energies to the IP 3 binding site in the crystal. Cluster size cannot be used for quantitative comparison between different ligands, however, it may suggest more plausible binding site for a given ligand. The cluster size at the IP 3 -binding site was the largest among any other clusters observed in this study ( Fig. 3a ), which might imply that the IP 3 is more likely to bind to the position found in the crystal. These data appeared to be consistent with the relatively strong binding of PI(4,5)P 2 to the ARD ( Fig. 1a ). 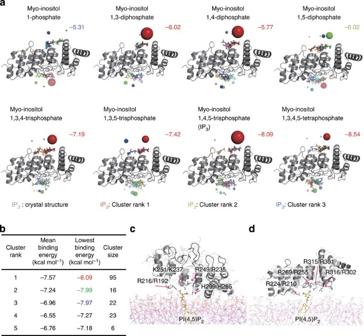Figure 3: Docking simulations between IP3and the TRPV4 ARD. (a) The binding modes of phosphorylated myo-inositols, the heads of phosphoinositides, to the TRPV4 ARD were predicted by AutoDock 4.2. The results are shown together with the IP3(grey) in the crystal. The lowest energy binding modes of the top ten clusters are represented by bubbles, corresponding to the size of the cluster. The size of the cluster is considered to roughly correlate with the possibility of binding. The estimated energy for the binding is also calculated (kcal mol−1). (b) The table presents the mean binding energies, the lowest binding energies and the sizes of the top five clusters in the docking of IP3to the ARD. Inaandb, the colour codes indicate the order of the cluster sizes. (c,d) Snapshots of the molecular dynamics simulations of the ARD with PI(4,5)P2-containing membranes. The binding of ARD on the surface was modelled, based on the IP3-binding site in the crystal (c) and the second binding site identified in the docking simulations (d). Figure 3: Docking simulations between IP 3 and the TRPV4 ARD. ( a ) The binding modes of phosphorylated myo-inositols, the heads of phosphoinositides, to the TRPV4 ARD were predicted by AutoDock 4.2. The results are shown together with the IP 3 (grey) in the crystal. The lowest energy binding modes of the top ten clusters are represented by bubbles, corresponding to the size of the cluster. The size of the cluster is considered to roughly correlate with the possibility of binding. The estimated energy for the binding is also calculated (kcal mol −1 ). ( b ) The table presents the mean binding energies, the lowest binding energies and the sizes of the top five clusters in the docking of IP 3 to the ARD. In a and b , the colour codes indicate the order of the cluster sizes. ( c , d ) Snapshots of the molecular dynamics simulations of the ARD with PI(4,5)P 2 -containing membranes. The binding of ARD on the surface was modelled, based on the IP 3 -binding site in the crystal ( c ) and the second binding site identified in the docking simulations ( d ). Full size image However, there are several clusters of IP 3 binding at the opposite side of the IP 3 binding site in the crystal of the ARD, although the sizes of the clusters are much smaller than that for the site in the crystal ( Fig. 3a,b ). Therefore, we tested the binding of the ARD on both surfaces of PI(4,5)P 2 -containing membranes in silico ( Fig. 3c,d ). The ARD was placed in either orientation, and the stability of the association to the membrane was examined. When the IP 3 -binding site in the crystal was placed on the membrane, the amino-acid residues, such as R216, K251, R249 and H299, were located in the proximity of PI(4,5)P 2 in silico , supporting the idea that the IP 3 -binding site in the crystal is also used as the PI(4,5)P 2 -binding site ( Fig. 3c ). However, when the ARD was placed with the opposite surface towards the membrane, the ARD was found to associate with the PI(4,5)P 2 -containing membrane in silico , where the amino-acid residues, such as R224, R269, R315 and R316, were located in the proximity of PI(4,5)P 2 ( Fig. 3d ). This surface is also positively charged ( Supplementary Fig. 4 ), and therefore, it might also be a potential membrane-binding site if the ARD is tethered to the membrane, which is the situation for a channel protein. Identification of amino-acid residues responsible for PI(4,5)P 2 binding in the TRPV4 ARD We then experimentally corroborated the IP 3 -binding site by a point mutation analysis. First, we tested the N296D-H299P human TRPV4 ARD mutant, in which two residues for interactions with P1 and P5, respectively, are mutated. H299 was substituted with proline, because the main chain NH interacted with P5 and the turn made by proline appeared to be identical to that made by H299 in the structure. The N296D-H299P mutant ARD showed weaker binding to liposomes containing PI(4,5)P 2 than the TRPV4 ARD ( Fig. 4a ), and the dissociation constant for the N296D-H299P mutant ARD was determined to be 163 μM ( r =0.989) by an SPR analysis ( Supplementary Fig. 1 ). Importantly, H299P alone was sufficient for the decrease in the binding. This result is reasonable because N296 appeared to interact with the P1 site of IP 3 , which is not usually involved in the binding of PI(4,5)P 2 to the binding protein. Consistently, the K344E mutation in the P1 site did not reduce PI(4,5)P 2 binding ( Fig. 4a ). Taken together, the interaction of IP 3 with P1 did not appear to be essential for IP 3 /PI(4,5)P 2 binding. On the other hand, the K251E mutant for the water-mediated interaction with P4 also did not reduce PI(4,5)P 2 binding ( Fig. 4a ). The R249E mutant for P4 was not expressed, presumably because R249 interacted with other amino-acid residues for proper protein folding. 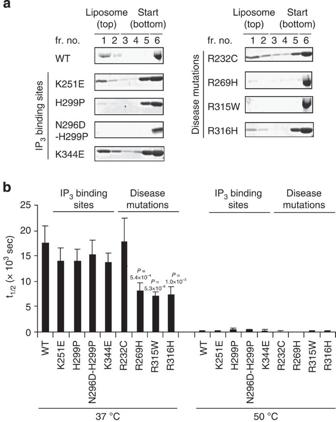Figure 4: PI(4,5)P2binding and stability of TRPV4 mutants. (a) Liposome floating assay. The binding of TRPV4 ARD (wild type: WT) and its mutants to PI(4,5)P2-containing liposomes was examined. Liposomes without PI(4,5)P2were used as a negative control for the TRPV4 ARD. The appearance of protein in the top fraction indicates a protein–lipid interaction. (b) Protein stability assay. The half-lives (t1/2) of the WT ARD and the mutants at 37 °C (physiological conditions) and 50 °C (denaturing conditions) were examined.Pvalues relative to WT are shown. Data points are mean±s.e.m. (n=3–6). Figure 4: PI(4,5)P 2 binding and stability of TRPV4 mutants. ( a ) Liposome floating assay. The binding of TRPV4 ARD (wild type: WT) and its mutants to PI(4,5)P 2 -containing liposomes was examined. Liposomes without PI(4,5)P 2 were used as a negative control for the TRPV4 ARD. The appearance of protein in the top fraction indicates a protein–lipid interaction. ( b ) Protein stability assay. The half-lives ( t 1/2 ) of the WT ARD and the mutants at 37 °C (physiological conditions) and 50 °C (denaturing conditions) were examined. P values relative to WT are shown. Data points are mean±s.e.m. ( n =3–6). Full size image We then examined the binding of the R232C, R269H, R315W and R316H mutants, identified in CMT2C and other diseases [7] , [8] , [9] , [25] . All of these mutants, except for R232C, showed significantly decreased binding to PI(4,5)P 2 -containing liposomes ( Fig. 4a ). The dissociation constant for the R315W mutant ARD was determined to be 232 μM ( r =0.876), which is much weaker than that of TRPV4 ARD, by an SPR analysis ( Supplementary Fig. 1 ). The R269/R255, R315/R301 and R316/R302 mutations are located on a different surface than the IP 3 -binding site in the crystal structure ( Fig. 2a ), but at a potential PI(4,5)P 2 -binding site in the docking simulation ( Fig. 3d ). However, the size of the cluster near the surface where the disease-associated mutations are located was smaller than that near the surface determined as an IP 3 -binding site by the crystal structure ( Fig. 3a,b ). Furthermore, the identification of the binding sites on the ARD by a docking simulation is not as reliable as compared with that identified by the crystal structure. Therefore, we explored another possibility, the protein unfolding, for the decreased PI(4,5)P 2 binding of the ARD because of the disease-associated mutations. The binding of dye to hydrophobic amino-acid residues was used to reveal protein unfolding. Importantly, the structure-based mutations at the IP 3 -binding site, H299P and N296D-H299P, did not affect the unfolding half-life ( Fig. 4b ). However, the R269H, R315W and R316H mutations destabilized the protein structure, as demonstrated by the shorter half-lives of these mutants than the wild-type (WT) ARD, as reported previously ( Fig. 4b ) [23] . In contrast, the R232C mutation did not destabilize the structure [23] . In the crystal structure, R269/R255 and R315/R301 form a salt bridge with D313/D299 and E286/E272, respectively ( Fig. 5a ). To confirm that the R269H and R315W mutations affect the protein stability, we performed molecular-dynamics simulations. We made the R269H or R315W mutation in the WT ARD in silico , and then the behaviours of the atoms were calculated for 100 ns. The mutations affected the distance between these pairs of amino-acid residues that form a salt bridge in the WT ARD ( Fig. 5b ). Therefore, the disease mutations are suggested to affect the overall structure of the ARD, from both the stability assay and molecular dynamics simulations. 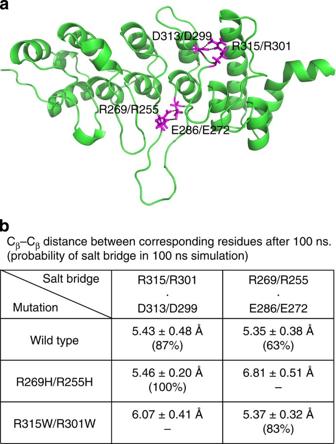Figure 5: Molecular-dynamics simulation of the R269H or R315W ARD mutants. (a) The salt bridges at R269 and R315. The interactions of R269 and R315 with the neighbouring amino-acid residues, E286 and D313, respectively. (b) The distances between R269 and E286, and R315 and D313 were calculated for 100 ns, and the results are shown in the table. Figure 5: Molecular-dynamics simulation of the R269H or R315W ARD mutants. ( a ) The salt bridges at R269 and R315. The interactions of R269 and R315 with the neighbouring amino-acid residues, E286 and D313, respectively. ( b ) The distances between R269 and E286, and R315 and D313 were calculated for 100 ns, and the results are shown in the table. Full size image Suppression of TRPV4 activity by PI(4,5)P 2 binding To explore the functional roles of phosphoinositides in the TRPV4 activity, we measured ionic currents in human embryonic kidney (HEK) 293 cells expressing human TRPV4 by whole-cell patch-clamp recording. Whole-cell currents evoked by the TRPV4 agonist, 4α-PDD [26] , were suppressed by adding PI(4,5)P 2 and to a somewhat lesser extent by adding PI(3,4,5)P 3 via a patch pipette solution ( Fig. 6a,b ). In contrast, PI(3,4)P 2 and PI(3,5)P 2 did not affect the TRPV4 activity. These sensitivities to phosphoinositides appeared to be consistent with the lipid-binding specificities ( Figs 1a and 3a ). As the concentration of PI(3,4,5)P 3 is generally assumed to be much lower than that of PI(4,5)P 2 , even in stimulated cells [27] , we focused on PI(4,5)P 2 and examined its effects on channel activities in detail. Interestingly, the onset of the current induced by 4α-PDD occurred earlier by the addition of PI(4,5)P 2 than that in its absence ( Supplementary Fig. 5 ). The manipulation of PI(4,5)P 2 appeared to work well, because the diffusion of PI(4,5)P 2 from the pipette into the cell and the increased PI(4,5)P 2 levels in the plasma membrane (PM) were confirmed by the fluorescently labelled BODIPY FL-labelled PI(4,5)P 2 and by the GFP-fused PH domain of PLC δ1 (PLCδ1PH), which binds specifically to PI(4,5)P 2 and IP 3 (refs 28 , 29; Supplementary Fig. 6 ). 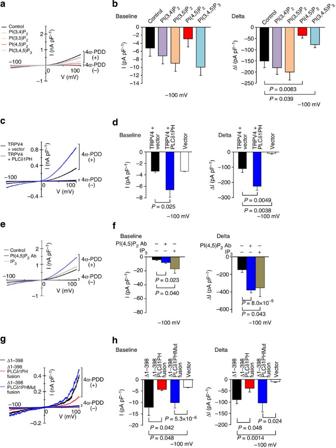Figure 6: Suppressed TRPV4 channel activity by PI(4,5)P2binding. (a) RepresentativeI–Vrelationships of whole-cell currents before and after exposure to 1 μM 4α-PDD in TRPV4-expressing HEK293 cells, dialyzed against 20 μM PI(3,4)P2, 20 μM PI(3,5)P2, 20 μM PI(4,5)P2or 20 μM PI(3,4,5)P3through a patch pipette. (b) Basal current densities and 4α-PDD-evoked current responses (ΔI) of TRPV4, in the presence of PI(3,4)P2, PI(3,5)P2, PI(4,5)P2or PI(3,4,5)P3, at −100 mV (n=6–12). (c) RepresentativeI–Vrelationships of whole-cell currents before and after exposure to 1 μM 4α-PDD in TRPV4-expressing HEK293 cells co-transfected with either an empty vector or the PLCδ1PH expression vector. (d) Basal current densities and 4α-PDD-evoked current responses (ΔI) of TRPV4 at −100 mV (n=7–9). (e) RepresentativeI–Vrelationships of whole-cell currents before and after exposure to 1 μM 4α-PDD in TRPV4-expressing HEK293 cells, dialyzed against 1% PI(4,5)P2antibody (PI(4,5)P2Ab) or 30 μM IP3through a patch pipette. (f) Basal current densities and 4α-PDD-evoked current responses of TRPV4 constructs, in the presence of PI(4,5)P2Ab or IP3at −100 mV (n=8–12). (g) RepresentativeI–Vrelationships of whole-cell currents before and after exposure to 1 μM 4α-PDD, in HEK293 cells expressing Δ1–398, Δ1–398 PLCδ1PH fusion or Δ1–398 PLCδ1PHMut fusion. (h) Basal current densities and 4α-PDD-evoked current responses of TRPV4 constructs at −100 mV (n=7–9). Data points are mean±s.e.m. Figure 6: Suppressed TRPV4 channel activity by PI(4,5)P 2 binding. ( a ) Representative I–V relationships of whole-cell currents before and after exposure to 1 μM 4α-PDD in TRPV4-expressing HEK293 cells, dialyzed against 20 μM PI(3,4)P 2 , 20 μM PI(3,5)P 2 , 20 μM PI(4,5)P 2 or 20 μM PI(3,4,5)P 3 through a patch pipette. ( b ) Basal current densities and 4α-PDD-evoked current responses (Δ I ) of TRPV4, in the presence of PI(3,4)P 2 , PI(3,5)P 2 , PI(4,5)P 2 or PI(3,4,5)P 3 , at −100 mV ( n =6–12). ( c ) Representative I–V relationships of whole-cell currents before and after exposure to 1 μM 4α-PDD in TRPV4-expressing HEK293 cells co-transfected with either an empty vector or the PLCδ1PH expression vector. ( d ) Basal current densities and 4α-PDD-evoked current responses (Δ I ) of TRPV4 at −100 mV ( n =7–9). ( e ) Representative I–V relationships of whole-cell currents before and after exposure to 1 μM 4α-PDD in TRPV4-expressing HEK293 cells, dialyzed against 1% PI(4,5)P 2 antibody (PI(4,5)P 2 Ab) or 30 μM IP 3 through a patch pipette. ( f ) Basal current densities and 4α-PDD-evoked current responses of TRPV4 constructs, in the presence of PI(4,5)P 2 Ab or IP 3 at −100 mV ( n =8–12). ( g ) Representative I–V relationships of whole-cell currents before and after exposure to 1 μM 4α-PDD, in HEK293 cells expressing Δ1–398, Δ1–398 PLCδ1PH fusion or Δ1–398 PLCδ1PHMut fusion. ( h ) Basal current densities and 4α-PDD-evoked current responses of TRPV4 constructs at −100 mV ( n =7–9). Data points are mean±s.e.m. Full size image To corroborate the suppressive effect of PI(4,5)P 2 on TRPV4 activity, we next decreased the PI(4,5)P 2 levels in the PM and examined the channel activities. The overexpression of the PLCδ1PH domain is thought to sequester PI(4,5)P 2 (and IP 3 , which exists at much lower levels than PI(4,5)P 2 in unstimulated cells) [29] , [30] . Consistently, the overexpression of the PLCδ1PH domain elevated the basal currents and the maximal currents upon 4α-PDD treatment ( Fig. 6c,d ). In addition, the basal currents and the maximal currents upon 4α-PDD treatment were increased by adding an anti-PI(4,5)P 2 antibody [31] or IP 3 through a patch pipette solution ( Fig. 6e,f ). Interestingly, the TRPV4 responses to 4α-PDD were slightly delayed by adding the PI(4,5)P 2 antibody or IP 3 ( Supplementary Fig. 5 ). The decreased levels of PI(4,5)P 2 in the PM by the addition of the anti-PI(4,5)P 2 antibody or IP 3 (ref. 29 ) were confirmed by GFP-PLCδ1PH ( Supplementary Fig. 6 ). Whole-cell currents evoked by hypo-osmotic and heat stresses [1] , [2] were also suppressed by adding PI(4,5)P 2 , but were enhanced by adding the PI(4,5)P 2 antibody or IP 3 in TRPV4-expressing HEK293 cells ( Supplementary Figs 7 and 8 ), indicating that PI(4,5)P 2 suppresses TRPV4 activities regardless of the type of stimuli. The positive effect of IP 3 on TRPV4 channel function was previously reported [32] . Considering that IP 3 is the head group of PI(4,5)P 2 , IP 3 may compete with PI(4,5)P 2 for ARD binding [33] . Consistent with this notion, 4α-PDD-evoked currents through TRPV4 were suppressed by the addition of the longer acyl chains of PI(4,5)P 2 (diC8-PI(4,5)P 2 and diC16-PI(4,5)P 2 ), but were augmented by the addition of the shorter acyl chains of PI(4,5)P 2 (diC4-PI(4,5)P 2 ) ( Supplementary Fig. 9 ). As the hydrophilicity of diC4-PI(4,5)P 2 is higher than those of diC8-PI(4,5)P 2 and diC16-PI(4,5)P 2 , diC4-PI(4,5)P 2 can be easily removed from the membrane, and may prevent ARD membrane association and increase the channel activity, in a similar manner to IP 3 . Finally, to examine the importance of PI(4,5)P 2 binding at the N-terminal region of TRPV4, we next deleted the N-terminal ARD (Δ1–398) or replaced it with PLCδ1PH (Δ1–398 PLCδ1PH fusion) or with a PLCδ1PH mutant bearing the R40D mutation [28] to diminish the interaction with PI(4,5)P 2 (Δ1–398 PLCδ1PH-Mut fusion), and compared the responses of these mutants to TRPV4 agonists ( Fig. 6g,h and Supplementary Fig. 10 ). These mutants showed similar localization patterns in the PM, but the expression levels in the PM were somewhat impaired in comparison to the full-length TRPV4, as revealed by total internal reflection fluorescence (TIRF) microscopy, which illuminates only the subcellular area from the surface to a depth of less than 100 nm from the surface of the coverslips, and by the biotinylation labelling method ( Supplementary Fig. 11 ). The Δ1–398 mutant was still able to elicit significant responses to 4α-PDD and hypo-osmotic stress, but not to heat stress, as previously reported [34] ( Fig. 6g,h and Supplementary Fig. 10b,c ). Notably, consistent with the idea of the suppression of TRPV4 by PI(4,5)P 2 binding at its N-terminus, the presence of the PH domain (Δ1–398 PLCδ1PH fusion mutant) diminished the TRPV4 responses to 4α-PDD and hypo-osmotic stress, whereas the PH-domain mutant (Δ1–398 PLCδ1PH-Mut fusion mutant) showed comparable channel activities to the Δ1–398 mutant ( Fig. 6g,h and Supplementary Fig. 10b,c ). Thus, PI(4,5)P 2 binding to the N-terminus of TRPV4 exerts an inhibitory effect on the channel activity. PI(4,5)P 2 insensitivity of disease-associated TRPV4 mutants We next measured the currents of TRPV4 mutants with impaired PI(4,5)P 2 binding. The R269H, N296D-H299P, H299P, R315W and R316H mutants, which showed impaired PI(4,5)P 2 binding ( Fig. 4a ), exhibited elevated basal activities and higher responses to TRPV4 agonists ( Fig. 7 and Supplementary Figs 7, 8 and 12 ). The enhanced activities of these mutants are not attributable to altered membrane expression, as the mutants showed intact PM expression similar to TRPV4 ( Supplementary Fig. 11 ). The suppressive effect of PI(4,5)P 2 and the augmentative effect of the PI(4,5)P 2 antibody and IP 3 on the TRPV4 activities were not observed with these mutants ( Fig. 7 and Supplementary Figs 7 and 8 ). In contrast, the R232C, K251E and K344E mutants, which showed PI(4,5)P 2 binding ( Fig. 4a ), responded to PI(4,5)P 2 , the PI(4,5)P 2 antibody and IP 3 ( Fig. 7 ). The whole-cell currents via the K251E and K344E mutants under basal and 4α-PDD-stimulated conditions were similar to those via TRPV4 ( Figs 6 and 7 ). The R232C mutant exhibited marginally increased currents, in spite of the decreased membrane expression ( Supplementary Fig. 11a ). Interestingly, R232C was localized in a dot-like structure in the PM, whereas TRPV4 and the other mutants were localized in filament-like structures in the PM ( Supplementary Fig. 11b ). 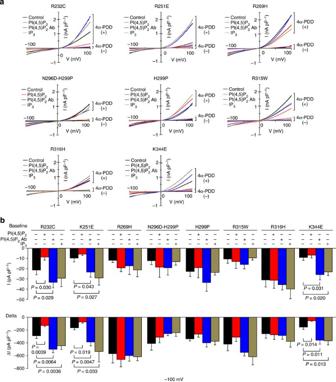Figure 7: PI(4,5)P2sensitivities of TRPV4 mutants. Effects of intracellular PI(4,5)P2and IP3on the activities of R232C, R251E, R269H, N296D-H299P, H299P, R315W, R316H and K344E. (a) RepresentativeI–Vrelationships of whole-cell currents before and after exposure to 1 μM 4α-PDD in TRPV4 construct-expressing HEK293 cells, dialyzed against 20 μM diC8-PI(4,5)P2, 1% PI(4,5)P2Ab or 30 μM IP3through a patch pipette. (b) Basal current densities and 4α-PDD-evoked current responses of TRPV4 constructs, in the presence of diC8-PI(4,5)P2, PI(4,5)P2Ab or IP3at −100 mV (n=5–17). Data points are mean±s.e.m. Figure 7: PI(4,5)P 2 sensitivities of TRPV4 mutants. Effects of intracellular PI(4,5)P 2 and IP 3 on the activities of R232C, R251E, R269H, N296D-H299P, H299P, R315W, R316H and K344E. ( a ) Representative I–V relationships of whole-cell currents before and after exposure to 1 μM 4α-PDD in TRPV4 construct-expressing HEK293 cells, dialyzed against 20 μM diC8-PI(4,5)P 2 , 1% PI(4,5)P 2 Ab or 30 μM IP 3 through a patch pipette. ( b ) Basal current densities and 4α-PDD-evoked current responses of TRPV4 constructs, in the presence of diC8-PI(4,5)P 2 , PI(4,5)P 2 Ab or IP 3 at −100 mV ( n =5–17). Data points are mean±s.e.m. Full size image Most patients suffering from TRPV4 channelopathies carry a normal TRPV4 and a mutant allele of TRPV4. We therefore examined the PI(4,5)P 2 sensitivity of TRPV4 currents with HEK293 cells co-expressing TRPV4 and the mutants ( Supplementary Fig. 13 ). HEK293 cells co-expressing TRPV4 and either the R269H, R315W or N296D-H299P mutant showed elevated basal activities and higher responses to 4α-PDD ( Supplementary Fig. 13b,c ). In addition, these currents were insensitive to PI(4,5)P 2 , the PI(4,5)P 2 antibody and IP 3 ( Supplementary Fig. 13b,c ). We immunoprecipitated TRPV4 with the co-expressed R269H, R315W or N296D-H299P mutant ( Supplementary Fig. 13a ), and the results suggested that hetero-multimeric channels may be causing the disease phenotype. To verify the functional impacts of PI(4,5)P 2 on the TRPV4 activity under physiological conditions, we measured Ca 2+ mobilization in HEK293 cells expressing TRPV4 or the mutants upon PLC activation, by stimulating G-protein-coupled receptors with ATP [32] . The 4α-PDD-induced Ca 2+ responses of TRPV4 were potentiated by 10 μM ATP ( Fig. 8a,b and Supplementary Fig. 14 ), suggesting that PI(4,5)P 2 hydrolysis by PLC increases the TRPV4 activity. Notably, ATP-induced enhancement of channel activity was not observed with the R269H, R315W and N296D-H299P mutants ( Fig. 8a,b and Supplementary Fig. 14 ), which instead showed elevated basal activities and enhanced responses to 4α-PDD in the absence of ATP ( Fig. 8a,b and Supplementary Fig. 14 ). Consistently, the overexpression of the PLCδ1PH domain [30] elevated the basal intracellular Ca 2+ concentration ([Ca 2+ ] i ), enhanced the Ca 2+ responses of TRPV4 to 4α-PDD, and suppressed the responses to ATP ( Fig. 8a,b and Supplementary Fig. 14 ). Under these conditions, both Ca 2+ influx through TRPV4 and Ca 2+ release from the endoplasmic reticulum in the presence of 10 μM ATP were negligible, as compared with the potentiating effect of the same concentration of ATP on 4α-PDD-induced Ca 2+ influx ( Supplementary Fig. 15 ). 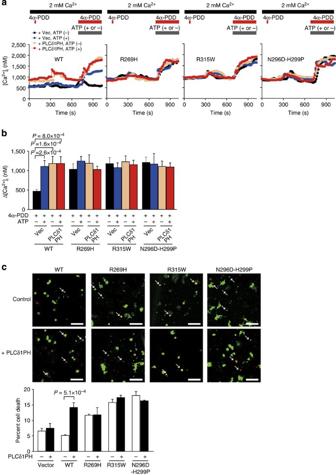Figure 8: Promoted TRPV4 activity and cell death by titration or hydrolysis of membrane PI(4,5)P2. (a,b) The effects of 10 μM ATP on 1 μM 4α-PDD-evoked [Ca2+]iresponses in TRPV4 construct-expressing HEK293 cells transfected with vector or PLCδ1PH. Averaged time courses (a) and maximal [Ca2+]iincreases (Δ[Ca2+]i) (b) in 4α-PDD-responding cells are shown (n=9–23). (c) Quantification of cell death in TRPV4 construct-expressing HEK293 cells transfected with a GFP-marker plasmid (pEGFP) together with vector or PLCδ1PH. Representative fluorescence images of propidium iodide (red) and GFP (green) and percent cell death are shown. Data are averaged from three independent experiments. The bar indicates 100 μm. Data points are mean±s.e.m. Figure 8: Promoted TRPV4 activity and cell death by titration or hydrolysis of membrane PI(4,5)P 2 . ( a , b ) The effects of 10 μM ATP on 1 μM 4α-PDD-evoked [Ca 2+ ] i responses in TRPV4 construct-expressing HEK293 cells transfected with vector or PLCδ1PH. Averaged time courses ( a ) and maximal [Ca 2+ ] i increases (Δ[Ca 2+ ] i ) ( b ) in 4α-PDD-responding cells are shown ( n =9–23). ( c ) Quantification of cell death in TRPV4 construct-expressing HEK293 cells transfected with a GFP-marker plasmid (pEGFP) together with vector or PLCδ1PH. Representative fluorescence images of propidium iodide (red) and GFP (green) and percent cell death are shown. Data are averaged from three independent experiments. The bar indicates 100 μm. Data points are mean±s.e.m. Full size image All of these results strongly support the conclusion that TRPV4 activities are suppressed through the ARD-PI(4,5)P 2 association, which upon perturbation causes TRPV4 to adopt a gain-of-function phenotype. Loss of PI(4,5)P 2 binding confers susceptibility to cell death Intracellular Ca 2+ signals are crucial for diverse cellular processes such as survival and death; therefore, cells expressing the TRPV4 mutants might struggle to maintain [Ca 2+ ] i at non-toxic levels. Indeed, propidium iodide uptake experiments revealed that the expression of the N296D-H299P mutant, as well as the R269H and R315W mutants [9] , [10] , caused a marked increase in cell death ( Fig. 8c ). Furthermore, the co-expression of PLCδ1PH with TRPV4 resulted in a remarkable increase in cell death, whereas co-expression with the TRPV4 mutants did not ( Fig. 8c ). These results suggested that defective PI(4,5)P 2 binding contributes to the increased activity of certain disease-associated TRPV4 mutants that cause cellular toxicity and increased cell death. In this study, we found that the TRPV4 ARD binds to phosphoinositides, especially PI(4,5)P 2 , which suppress TRPV4 activities. TRPV4 channel activities and cell death were increased by the hydrolysis of membrane PI(4,5)P 2 . Site-directed mutagenesis of the PI(4,5)P 2 -binding residues, identified in the ARD·IP 3 structure, increased the TRPV4 channel activities and cell death. These findings demonstrated that the loss of PI(4,5)P 2 binding results in increased TRPV4 activities and elevated cell death. Notably, the disease-associated R269H, R315W and R316H mutations abolished the PI(4,5)P 2 binding and PI(4,5)P 2 sensitivity. Thus, defective PI(4,5)P 2 binding to the TRPV4 ARD and consequent intracellular cation/Ca 2+ deregulation might contribute to cellular toxicity in some diseases, including CMT2C, CDSMA and SPSMA. The suppressive effect of PI(4,5)P 2 on TRPV4 activity is reasonable, in the context of the intracellular signalling events that regulate TRPV4 activities. PI(4,5)P 2 hydrolysis by PLC produces IP 3 , which sensitizes TRPV4 activity [32] , and DAG. The sensitizing effect of IP 3 is considered to be mediated by the association between TRPV4 and IP 3 receptor [32] , although the detailed mechanisms remain elusive. Our findings of direct binding of IP 3 and PI(4,5)P 2 to the TRPV4 ARD and the loss of channel regulation by PI(4,5)P 2 and IP 3 in mutants at the IP 3 -binding site suggested that IP 3 competes with PI(4,5)P 2 for ARD binding, to relieve TRPV4 inhibition. With regard to DAG, it is proposed to stimulate AA synthesis through the activation of protein kinase C [35] , [36] and is further metabolized to a TRPV4 agonist AA by DAG lipase [37] . Therefore, DAG also might exert a positive effect on the TRPV4 activity. However, the level of AA production induced by DAG appeared to be insufficient to increase the TRPV4 activities, at least under our experimental conditions, because 1-oleoyl-2-acetyl-sn-glycerol, a membrane-permeable DAG analogue, neither activated TRPV4 directly nor enhanced the 4α-PDD-stimulated responses of TRPV4 ( Supplementary Fig. 16 ). Therefore, the observed enhancement of TRPV4 activity by ATP receptor stimulation ( Fig. 8a,b ) is thought to be achieved by decreasing PI(4,5)P 2 and by increasing IP 3 production, but not by producing DAG. It will be interesting to explore further the functional coupling between the PLC-PI(4,5)P 2 hydrolysis-IP 3 and PLA 2 -AA-EET pathways, in the context of TRPV4 activation. The onset of TRPV4 responses to 4α-PDD was somewhat accelerated by adding PI(4,5)P 2 , in spite of the dramatic decrease in the total changes of current densities ( Supplementary Fig. 5 ). Interestingly, such a change in the kinetics of the TRPV4 currents has also been shown for a change in the extracellular Ca 2+ concentration [38] , [39] . TRPV4 responses to 4α-PDD were reported to be accelerated but rapidly decayed, and the amplitudes of the evoked currents were small at high extracellular Ca 2+ concentrations, whereas the amplitudes increased and the decay was markedly delayed at lower Ca 2+ concentrations [38] , [39] . Therefore, PI(4,5)P 2 and Ca 2+ may play multiple functional roles, probably in an activation state-dependent manner. Recently, the high-resolution structure of tetrameric TRPV1 was reported [40] , [41] . In this structure, the TRPV1 ARD appeared to be located apart from the membrane. However, our molecular dynamics simulation study implied that the PI(4,5)P 2 could reach and interact with the ARD of TRPV1 ( Supplementary Fig. 17 ). The TRPV1 structures reported by Liao et al. and Cao et al. were solved in lipids without PI(4,5)P 2 . PI(4,5)P 2 generally has longer acyl-chains, and thus its head group might be able to come closer to the binding site in the ARD than those of other lipids. When the TRPV4 ARD was superimposed on the full-length TRPV1 structure, the IP 3 -binding site faced the cytoplasm, and did not overlap with the contact site of the linker region that connects each subunit ( Supplementary Fig. 18 ). However, our data, including the experiments with the mutant TRPV4 where the ARD was substituted with the PH domain of PLCδ1, which specifically binds to PI(4,5)P 2 , supported the suppressive role of PI(4,5)P 2 binding to the ARD. We therefore speculate that the geometry of the TRPV4 ARD might be slightly but significantly different from that of the TRPV1 ARD in the full-length structure embedded in the PI(4,5)P 2 -containing membrane. This hypothesis is supported by lines of evidence from structural and functional points of view. The cryo-electron microscopic studies of TRPV1 indicated the relatively vertical orientation of the ARD, whereas those for TRPV4 suggested that the ARD sat on the membrane in an oblique orientation [4] , [42] . Notably, amino-acid residues 404–407 of rat TRPV1, which are located in the linker region between the ARD and transmembrane region, are not conserved in the human TRPV4. In particular, the counterpart of P407 in the rat TRPV1 is E444 in the human TRPV4. A proline residue creates a structural constraint, because its side chain cyclizes back to the backbone amide. Considering that Pro407 is located immediately beneath the pre-transmembrane S1 helix [43] , it is reasonable to suppose that Pro407 may determine the angle and flexibility of the N-terminal cytoplasmic region, including the TRPV1 ARD. The importance of the linker region in the TRPV4 function has been demonstrated, using a TRPV4 variant lacking the linker region [43] . With regard to the structure of the ARD, positively charged amino acids (Lys, Arg and so on) are clustered at and near the binding site for the head group of PI(4,5)P 2 in TRPV4, whereas they are not concentrated in the corresponding area of TRPV1 ( Supplementary Fig. 4 ). This suggests that the positively charged cluster of the TRPV4 ARD stabilizes the binding site of the ARD on the surface of the PI(4,5)P 2 -containing membrane. It must be noted that the regulatory factors of the TRPV4 channels (activation triggers, inhibitors and interacting proteins) are very different from those of the TRPV1 channels. Thus, the structural characteristics of TRPV4 are not completely comparable with those of TRPV1, but have rather diverged. Alternatively, it is possible that the other surface of the TRPV4 ARD might interact with the negatively charged membrane including PI(4,5)P 2 . To assess this idea, we ran the molecular-dynamics simulation and found that the ARD placed on the membrane with the opposite surface also appear to stably associate with it. Interestingly, the association on this ‘opposite’ surface is mediated by the amino-acid residues that are mutated in diseases ( Fig. 3d ). In addition, TRPV4 has a sequence of consecutive basic amino-acid stretches within the N-terminal tail [44] , which could function as a binding site for acidic lipids. In these cases, IP 3 , which is diffusible, might bind to both the PI(4,5)P 2 -binding and IP 3 -binding sites. This could not only relieve TRPV4 from inhibition by PI(4,5)P 2 but also induce global conformational changes in the TRPV4 protein, through neutralization of the surface charge to directly affect the channel activity, although the isolated ARD structure itself was not largely influenced by IP 3 binding ( Fig. 2d ). Another possibility is that the TRPV4 protein is inserted into the PM as a monomeric form through the interaction between PI(4,5)P 2 and the ARD. Given this situation, the TRPV4 proteins might only form a functional tetrameric channel after the hydrolysis or sequencing of PI(4,5)P 2 . Furthermore, we cannot exclude the possibility that the TRPV4 ARD interacts with PI(4,5)P 2 localized in the inner membrane [45] . Thus, the structural basis of the PI(4,5)P 2 -induced suppression of TRPV4 channel activities is still unknown. To understand it, further studies, including the determination of the high-resolution structure of TRPV4, are needed. If the IP 3 -binding surface determined by our crystallographic study faces the membrane, then the reason for the lack of PI(4,5)P 2 binding by the disease mutants, such as R269H, R315W and R316H, may result from the destabilization of the overall protein structure, as shown in Figs 4 and 5 . Given this situation, we cannot exclude the possibility that the gain-of-function phenotype of these mutants is attributable to an alteration in interactions with other regulatory factors, caused by protein instability. Indeed, the loss of ATP binding becasuse of protein instability has been reported for the R269H mutant protein [23] , although there is no correlation between the disease phenotype and the ATP binding, as intracellular ATP sensitizes TRPV4 activities [39] . However, the H299P and N296D-H299P mutants, which carry one or more mutation(s) in the IP 3 -binding site determined by our crystallographic study, retained intact protein stability ( Fig. 4b ), indicating that the decreased PI(4,5)P 2 binding results in the loss of PI(4,5)P 2 -mediated channel regulation and the augmentation of channel activity. This finding strongly suggests that the gain-of-function phenotypes of the R269H, R315W and R316H mutants are at least in part becasuse of decreased PI(4,5)P 2 binding. To clarify this, further identification of regulatory factors and their relationships to the PI(4,5)P 2 binding will be necessary. Among the disease-associated ARD mutations we tested, only the R232C mutation did not affect the PI(4,5)P 2 sensitivity and protein stability. This implies that the R232C mutation elicits a gain-of-function phenotype through PI(4,5)P 2 -independent mechanisms. Interestingly, the R232C mutant was localized in a dot-like structure in the PM, in contrast to the localization of TRPV4 and its mutants bearing the R269H, R315W or R316H mutation in filament-like structures ( Supplementary Fig. 11b ). Therefore, the R232C mutation may disrupt the association with cytoskeletal proteins, such as microfilament-associated protein 7 (ref. 46 ). Alternatively, the N-terminus of TRPV4 (amino-acid residues 40–235) is known to interact with OS-9, which facilitates the proper folding of TRPV4 and further tetramer formation in the endoplasmic reticulum [47] , suggesting the involvement of OS-9 in the CMT2C phenotype of R232C. Therefore, the molecular pathogenesis of the R232C mutation will be an interesting subject for future studies. In spite of our data suggesting the PI(4,5)P 2 -mediated regulation of TRPV4, the pathogenesis of diseases with TRPV4 mutations can be induced by other malfunctions besides the defective PI(4,5)P 2 binding at the ARD, as suggested by the R232C mutation. A large number of other dominant missense TRPV4 mutations outside the ARD have been identified in diverse hereditary diseases [1] . For example, the P799R or T701I mutation has been reported for various diseases, including CMT2C, CDSMA and SPSMA, although it remains unknown whether these mutations elicit a gain-of-function phenotype [1] . However, it should be noted that the majority of the CMT2C-, CDSMA- and SPSMA-associated mutants that are known to exhibit a gain-of-function phenotype showed impaired PI(4,5)P 2 sensitivity, which establishes a correlation between the PI(4,5)P 2 sensitivity and the disease phenotype. To obtain direct evidence of the significance of the defective PI(4,5)P 2 binding in the diseases, generation and characterization of knock-in mice carrying a mutation in PI(4,5)P 2 -binding domain of TRPV4 will be necessary. Recently, Garcia-Elias et al. reported that PI(4,5)P 2 facilitates TRPV4 responses to hypo-osmotic and heat stresses [44] . Interestingly, our results showed that the TRPV4 responses to 4α-PDD are slightly enhanced by PI(4,5)P 2 during the first 20 s after the application of the stimuli ( Supplementary Fig. 5 ). It is possible that the TRPV4 currents occurring only immediately after the treatment with stimuli were observed in the previous study. In addition, the effects of diC8-PI(4,5)P 2 were assessed by different experimental methods: excised patch measurements in the previous study and the whole-cell configuration in the present study. As intracellular factors are lost in excised patch measurements, it is also possible that some other factors and PI(4,5)P 2 might cumulatively influence TRPV4 activities in intact cells. The present study is the first demonstration of the lipid-binding ability of the ARD. Basically, phosphoinositide-binding proteins show two types of binding mode: ‘non-specific’ electrostatic complementarity and specific binding to particular headgroups [13] , [14] , [15] , [48] . The ‘non-specific’ binding occurs with the cluster of basic-charged amino-acid residues to acidic phosphoinositides, which can be observed with both unstructured stretches of basic-charged amino-acid residues, such as of N-WASP and small GTPases, and structured fold, such as of BAR domains. The specific binding occurs with PH domains, FYVE domains, C2 domains and several other domains, which have binding pockets for particular phospholipids. As we have shown here, ARDs appear to adapt both modes of interactions to phosphoinositides. It is possible that the lipid-binding ability is shared by some other ARDs. The ARD is present in more than 500 human proteins, with diverse binding specificities and affinities [49] . This characteristic of ARDs is thought to be based on the high diversity of their surfaces, because of various numbers and combinations of ankyrin repeats [50] . Consistently, artificial ankyrin repeat proteins (DARpin) can be selected for targeting to specific proteins from a library of artificial ARDs, but have not been rationally designed [51] . This characteristic of ARDs is comparable to that of antibodies, in that antibodies can be generated against lipids, including PI(4,5)P 2 (ref. 52 ). Therefore, the highly diverse characteristics of ARDs may support their ability to recognize a variety of molecules, including lipids. Preparation of the TRPV ARD protein The gene encoding the chicken TRPV4 ARD (residues 133–382) was cloned into the Nde I and Sal I sites of the pET22b vector (Novagen) with a C-terminal His 6 tag for crystallization. The Escherichia coli strain Rosetta 2 (DE3) (Stratagene) was transformed with the expression plasmid, and the cells were cultured in LB medium. The protein was overexpressed by induction with 1 mM isopropyl β- D -1-thiogalactopyranoside overnight at 20 °C. The collected cells were suspended in lysis buffer (20 mM Tris-HCl (pH 8.0), 300 mM NaCl, 20 mM imidazole (pH 8.0) and 1 mM phenylmethylsulfonyl fluoride), containing 0.1% Triton X-100, 0.2 mg ml −1 lysozyme, 50 μg ml −1 RNase A and 25 μg ml −1 DNase I, and were disrupted with an ultrasonic homogenizer. After centrifugation, the supernatant of the lysate was loaded onto a Ni Sepharose 6 Fast Flow column (GE Healthcare), which was eluted with 50 and 200 mM imidazole (pH 8.0) in lysis buffer. The fraction containing the protein was dialyzed against 20 mM Tris–HCl buffer (pH 8.0), containing 70 mM NaCl, 1 mM dithiothreitol (DTT) and 10% glycerol, and was loaded onto a Resource S column (GE Healthcare). The protein was eluted with a linear gradient of 0–2 M NaCl. The purified protein was further dialyzed against 20 mM Tris–HCl buffer (pH 8.0), containing 300 mM NaCl, 1 mM DTT and 10% glycerol, and was concentrated to 10.5 mg ml −1 . For the binding assays to liposomes, the WT or mutants of the human TRPV1 or TRPV4 ARD were expressed as glutathione- S -transferase fusion proteins, using the pGEX6P-1 vector (GE Healthcare). The proteins were then purified and the glutathione- S -transferase was removed by Prescission protease digestion. Liposome-binding assay The binding of the TRPV1 and TRPV4 ARDs to phosphoinositide-containing liposomes was examined by a co-sedimentation assay. The liposomes contained phosphatidylcholine, phosphatidylethanolamine, cholesterol, phosphoinositides and rhodamine-labelled PE (Avanti Polar Lipids), in a weight ratio of 10:2:8:2:0.7. Rhodamine-PE was incorporated to facilitate visualiztion of the liposome fraction. The lipids were first dissolved in chloroform/methanol/1 N HCl (80:80:1) for phosphoinositides or chloroform/methanol (1:1) for other lipids, mixed and dried under nitrogen gas, followed by under vacuum. The dried lipids were re-suspended to form liposomes for 1 h at 37 °C at a concentration of 2 μg μl −1 (total lipid) in Tris-buffered saline (TBS), containing 10 mM Tris–HCl (pH 7.5) and 150 mM NaCl, and subjected to five cycles of freezing (liquid N 2 ) and thawing (37 °C water bath). The ARD protein (0.5 μg μl −1 ) and liposomes (1 μg μl −1 ) were mixed in buffer containing 10 mM Tris-HCl (pH 7.5), 150 mM NaCl, 1 mM EDTA and 5% glycerol. After a 25-min incubation at room temperature, the liposomes were precipitated by centrifugation at 100,000 r.p.m. for 30 min in a TLA100 rotor (Beckman Coulter). The pellet and supernatant were examined by SDS–polyacrylamide gel electrophoresis (SDS–PAGE), and visualized by Simply Blue stain (Invitrogen), which is equivalent to Coomassie Brilliant Blue staining ( Supplementary Fig. 19 ). Representative data from three independent experiments are shown in the figure. The binding of the TRPV1 and TRPV4 ARDs to liposomes was examined by a floating assay, because of the instability of the TRPV4 ARD at a physiological ionic concentration. The liposomes contained phosphatidylcholine, phosphatidylethanolamine, cholesterol, PI(4,5)P 2 and rhodamine-PE, in a weight ratio of 10:2:8:0.7:0.25. The ARD protein (0.5 μg μl −1 ) and liposomes (1 μg μl −1 ) were mixed in TBS containing 10% glycerol and 40% Nycodenz/Histodenz (Sigma), and incubated for 15 min at room temperature. A 200-μl aliquot of the mixture was overlaid with 350 μl TBS containing 10% glycerol and 30% Nycodenz/Histodenz, followed by 70 μl TBS containing 10% glycerol. The layered solutions were then centrifuged at 48,000 r.p.m. for 4 h in an SW50 rotor (Beckman Coulter). The liposomes rose to the top, and fractions (100 μl each) were analyzed by SDS–PAGE. SPR experiments with nanodiscs containing PI(4,5)P 2 membrane Membrane scaffold protein (MSP) D1 is known to wrap lipid membranes into small particles. These particles containing lipid membranes are called ‘nanodiscs’, and are thought to behave like soluble molecules. Thus, nanodiscs can be used to measure lipid–protein interactions in solution [53] . To prepare nanodiscs, the MSP1D1 protein was expressed and purified as described previously [53] . 1-Palmitoyl-2-oleoylphosphatidylcholine (POPC) and PI(4,5)P 2 were solubilized in 100 mM cholate in ND buffer (20 mM Tris−HCl (pH 7.4), 100 mM NaCl) to final concentrations of 50 and 1.27 mM, respectively. The MSP1D1 protein was added in a molar ratio of MSP1D1:POPC:PI(4,5)P 2 =1:80:0 or 1:70:10. The lipid–protein mixture was gently rotated for 30 min at 28 °C. Subsequently, 0.8 g ml −1 of BioBeads SM-2 (Bio-Rad) equilibrated with ND buffer was added to 100 μl of the protein–lipid mixture to remove the cholate, and the suspension was placed on an orbital shaker for 1 h at 28 °C. The beads were removed by sedimentation, and the supernatant was dialyzed against ND buffer for 12 h. The nanodiscs after dialysis were purified by gel filtration on Superdex 200 10/300 (GE Healthcare), using SPR running buffer (10 mM HEPES (pH 7.5), 150 mM NaCl, 3 mM EDTA). In the final step, the nanodiscs were concentrated with an Amicon Ultra 10K filter (Merck Millipore). SPR-binding assays were performed at 25 °C on a BIAcore 2000 (GE Healthcare). BSA, chicken TRPV4 ARD, chicken TRPV4 R301W and chicken TRPV4 N282D-H285P were coupled to a sensor chip CM5 (GE Healthcare) by amine coupling. Binding analyses were performed at a flow rate of 5 μl min −1 , using a buffer containing 10 mM HEPES (pH 7.5), 150 mM NaCl and 3 mM EDTA. Each run consisted of consecutive injections of analyte (PI(4,5)P 2 -incorporated nanodiscs). The association and dissociation phases were measured for 7 and 5 min, respectively. Binding was examined at three different protein concentrations. The signals (response unit) were increased if the binding between nanodiscs and TRPV4 occurred in a concentration-dependent manner. This concentration-dependent increase was observed with PI(4,5)P 2 containing nanodiscs, but not with nanodiscs lacking PI(4,5)P 2 . Therefore, K d (= k diss / k ass ) values were successfully calculated from curve fitting only for PI(4,5)P 2 -containing nanodiscs. The apparent parameter for association ( k on ) dependent on the concentration was plotted, and the slope and the intercept of k on yielded k ass and k diss values, respectively. The measurement was evaluated with a correlation co-efficient for the fitting. Crystallization, IP 3 soaking and diffraction data collection The sitting drop vapour diffusion method was used for crystallization. Diffraction-quality crystals were obtained at 4 °C, by mixing 1 μl of protein solution and 1 μl of reservoir solution containing 110–120 mM sodium MES-HCl buffer (pH 6.5), 1–2% polyethylene glycol 4000, 11–12% 2-methyl-2,4-pentanediol and 55–60 mM KH 2 PO 4 . Crystals were transferred to the cryo-protective solution (50 mM sodium MES-HCl buffer (pH 6.5), 6.0% polyethylene glycol 4000, 12% 2-methyl-2,4-pentanediol, 10% glycerol and 100 mM NaCl) and flash-cooled at 90 K. For IP 3 soaking, crystals were transferred to the cryo-protective solution containing 10 mM IP 3 and incubated at 4 °C for 50 min, before flash-cooling. The diffraction data sets were collected at 90 K at the Photon Factory NW12A (Tsukuba) using a wavelength of 1.0000 Å. The data sets were processed using the HKL2000 programme [54] ( Table 1 ). Structure determination and refinement The crystal structures of the chicken TRPV4 ARD (with and without IP 3 ) were solved by the molecular replacement method with the Phaser programme [55] , using the coordinates of the reported chicken TRPV4 ARD structure (PDB ID: 3JXI [9] ) as the search model. The structure was refined against the data by iterative cycles of positional and temperature-factor refinements with the Phenix programme [56] and manual model building and revision with the Coot programme [57] . The same reflections were selected as the test-set reflections (2% of the data) for refinement of the crystal structures with and without IP 3 . The model of IP 3 was not included in the earlier stage of the refinement. It was placed in the corresponding intense F O − F C electron density map in later rounds. Several rounds of refinement after picking water molecules allowed the conversion of the R factors ( Table 1 ). In the final model of the IP 3 complex, 97.1% of all residues were in the preferred regions of the Ramachandran plot, 2.4% were in the allowed regions and 0.5% were outliers based on the validation in the Coot programme. In the structure without IP 3 , 96.1% were in the preferred regions, 3.5% were in the allowed regions and 0.4% were outliers. Docking simulation The binding modes of phosphorylated myo-inositols to the ARD were predicted with the molecular docking software, AutoDock4.2 (ref. 58 ). A total of 250 independent docking simulations were performed for each myo-inositol, and the 250 binding modes thus obtained were clustered into 27–41 clusters with 2.0 Å criterion. The lowest energy binding modes of the top ten clusters are shown in Fig. 3 . The location of IP 3 in the top cluster, which consists of 95 out of the 250 predicted structures (40%), is very close to that in the X-ray crystal structure (coloured grey in Fig. 3 ), validating the location of IP 3 determined in this study. Molecular dynamics simulation Simulation systems for the WT and two mutants, R255H and R301W, of ARD in TRPV4 in solution (total ~43,000 atoms including water and ions) were prepared, based on the crystal structure obtained in this study, and simulated for 100-ns. Modelling of the PI(4,5)P 2 -bound ARD with membrane was initiated by the generation of an equilibrated lipid bilayer system containing 288 diarachidonyl phosphatidyl choline (DAPC) molecules. Then, one of the DAPC head groups was replaced by PI(4,5)P 2 . Two models were generated, by setting the relative positions of PI(4,5)P 2 to the ARD identical with the crystal structure in this study or to the second-best binding mode in the docking simulations. Simulations of both systems (total ~145,000 atoms) were conducted for 100 ns under semi-isotropic pressure control, in which the pressure along the membrane normal is independent of the pressures along the other directions. To set up the simulation system of the TRPV1 tetramer in the membrane, the TRPV1 tetramer (PDB ID: 3J5P [40] , [41] ) was superimposed on an equilibrated lipid bilayer system in solution containing 648 DAPC, so that the centre of mass of the TRPV1 transmembrane region fit with that of the lipid bilayer. Subsequently, 182 DAPCs and solvent molecules that overlapped with the TRPV1 tetramer were removed. Twenty head groups of DAPC in each leaflet were randomly selected and replaced with PI(4,5)P 2 . The 200-ns simulations (~350,000 atoms) were performed, using the aforementioned semi-isotropic pressure control. All of the molecular dynamics simulations were performed using NAMD 2.9 (ref. 59 ), employing periodic boxes with gaps filled with water and 150 mM KCl. The CHARMM 22 (ref. 60 ) force field with CMAP [61] was used for the protein and KCl, and the TIP3P (CHARMM) model was used for water molecules. The CHARMM 36 force field for lipids [62] was employed for DAPC and the tail group of PI(4,5)P 2 , and that for carbonyl [63] was used for the PI(4,5)P 2 head group. The bond, angle and dihedral parameters of the atoms that connect the phosphorylated inositol and the tail group were obtained from the lipid parameters. The systems were brought to thermodynamic equilibrium at 300 K and 1 atm, using a Langevin thermostat and barostat. Equations of motion were integrated with a time step of 2 fs. The long-range Coulomb energy was evaluated using the particle mesh Ewald method. Protein stability assay The stability of the TRPV4 ARD protein (3.6 mg ml −1 , in 20 mM Tris-HCl buffer (pH 8.0) containing 300 mM NaCl, 1 mM DTT and 10% glycerol) was monitored by a dye-binding assay [64] . The PSA dye (PSA200K; ProFoldin) was used according to the manufacturer’s instructions, at 37 °C (physiological conditions) or 50 °C (denaturing conditions), with excitation at 550 nm and emission monitored at 610 nm, using a spectrofluorometer (FP6500; JASCO). The half-lives of the proteins were calculated using the following curve fitting formula: F =FN+[FU × t/(t 1/2 +t)], where t is the incubation time of the protein at the selected temperature; F is the fluorescence of the sample at time t ; FN is the fluorescence of the unheated sample ( t =0); t 1/2 is the half-life and FU is the maximum fluorescence of the curve representing the fluorescence of the completely unfolded protein at the plateau. The data from more than five experiments are shown, together with the standard error of the mean (s.e.m.). Plasmid construction for expression in mammalian cells Human TRPV4 (hTRPV4) was C-terminally tagged with mCherry, by inserting the hTRPV4 gene into the pmCherry-N3 vector, in which the EGFP in the pEGFP-N3 vector (Clontech) was replaced with mCherry. Amino-acid substitutions were introduced with a QuikChange mutagenesis kit (Stratagene). The Δ1–398 mutant, tagged with EGFP at the N-terminus, was inserted into the pmCherry-N3 vector. The PLCδ1 PH domain and the R40D PLCδ1 PH domain, in which the amino-acid responsible for PI(4,5)P 2 binding is mutated [28] , were inserted between EGFP and Δ1–398, to construct the Δ1–398 PLCδ1 PH fusion and the Δ1–398 PLCδ1 PHMut fusion, respectively. Cell culture and cDNA expression HEK293 cells were cultured in Dulbecco’s modified Eagle’s medium containing 10% fetal bovine serum, 30 U ml −1 penicillin and 30 μg ml −1 streptomycin, under a 95% air-5% CO 2 atmosphere at 37 °C. For the electrophysiological and [Ca 2+ ] i measurements and the cell death assay, HEK293 cells were co-transfected with recombinant plasmids and pEGFP-F (Clontech) as a transfection marker, using the SuperFect Transfection Reagent (Qiagen). HEK293 cells were plated onto poly- L -lysine-coated glass coverslips 24 h after transfection, and were subjected to electrophysiological and [Ca 2+ ] i measurements, cell surface labelling experiments, TIRF imaging, co-immunoprecipitation assays and cell death assays 8–30 h afterwards. Electrophysiology Currents from cells were recorded at room temperature (22–25 °C), using whole-cell mode patch-clamp techniques with an EPC-9 patch-clamp amplifier (Heka Electronics), as previously described [65] . The patch electrodes were prepared from borosilicate glass capillaries and had a resistance of 2–4 MΩ. Current signals were filtered at 5 kHz with a four-pole Bessel filter and digitized at 10 kHz. The PatchMaster (Heka Electronics) software was used for command pulse control, as well as data acquisition and analysis. Series resistance was compensated (to 70–80%) to minimize voltage errors. The cells were maintained at −30 mV, and the currents were elicited by slow voltage ramps (from −100 mV to +100 mV, 0.6 s duration). The standard extracellular (bath) solution contained 100 mM NaCl, 6 mM KCl, 2 mM MgCl 2 , 1.5 mM CaCl 2 , 10 mM glucose and 10 mM HEPES (pH 7.38 adjusted with NaOH, and osmolality adjusted to 300 mmol kg −1 with sucrose) [7] . The standard intracellular (pipette) solution contained 140 mM CsCl, 2 mM MgCl 2 , 10 mM EGTA, 2 mM Na 2 ATP, 0.1 mM NaGTP and 10 mM HEPES (pH 7.28 adjusted with CsOH, and osmolality adjusted to 298 mmol kg −1 with sucrose) [7] . For hypo-osmotic stress, we superfused cells with a solution containing 95 mM NaCl, 6 mM CsCl, 1 mM MgCl 2 , 1.5 mM CaCl 2 , 10 mM glucose and 10 mM HEPES (pH 7.38 adjusted with NaOH, and osmolality adjusted to 210 mmol kg −1 with sucrose) [66] . Iso-osmolarity was achieved by adding sucrose to this solution to reach 315 mmol kg −1 . The intracellular (pipette) solution contained 20 mM CsCl, 100 mM aspartate, 1 mM MgCl 2 , 4 mM Na 2 ATP, 10 mM BAPTA, 2.93 mM CaCl 2 and 10 mM HEPES (pH 7.28 adjusted with CsOH, and osmolality adjusted to 300 mmol kg −1 with sucrose) [66] . The free Ca 2+ concentration of this solution was 50 nM. To prevent activation of the volume-regulated anion current, the cells were dialyzed with a pipette solution containing 10 mM BAPTA [67] . These pipette solutions also contained diC4-PI(4,5)P 2 (Echelon Biosciences); diC8-PI(4,5)P 2 (Echelon Biosciences); diC16-PI(4,5)P 2 (Echelon Biosciences); diC16-PI(3,4)P 2 (Echelon Biosciences); diC8-PI(3,5)P 2 (Echelon Biosciences); diC8-PI(3,4,5)P 3 (Echelon Biosciences); BODIPY FL-labelled PI(4,5)P 2 (Echelon Biosciences); a mouse monoclonal PI(4,5)P 2 antibody (Abcam, dialyzed with Slide-A-Lyzer Dialysis Cassettes 10K MWCO, Thermo Fisher Scientific) or IP 3 (Dojindo). Multiply-phosphorylated phosphoinositides were stored as 2 mM stock solutions in the intracellular solution and sonicated before use. Unless otherwise indicated, diC8-PI(4,5)P 2 was used to mimic the endogenous PI(4,5)P 2 . Recording of currents was started at least 5 min after membrane rupture, to allow the compounds applied through the patch pipette to diffuse throughout the entire cell ( Supplementary Fig. 6 ) [31] , [68] . The 4α-PDD or hypo-osmotic stress-evoked currents were obtained by subtracting the basal density of the whole cell inward currents from that recorded under 4α-PDD treatment or hypo-osmotic stress at –100 mV. Cell surface labelling experiment The cell surface expressions of GFP-tagged TRPV4 constructs were measured by biotinylation, as previously described [65] with modifications. The cells were incubated with 0.5 mg ml −1 Sulfo-NHS-SS-Biotin (Thermo Scientific) in PBS for 30 min at 4 °C. The cells were washed with PBS containing 100 mM glycine three times, to stop the biotinylation reaction and to remove the free biotin. The cells were then lysed in RIPA buffer (pH 8.0) containing 150 mM NaCl, 1% Nonidet P-40, 0.5% sodium deoxycholate, 0.1% SDS and 50 mM Tris. After centrifugation, the supernatant was collected and incubated with streptavidin-agarose beads (Thermo Scientific) for 2 h at 4 °C. The beads were washed with RIPA buffer six times. The proteins were eluted in SDS sample buffer containing 50 mM DTT, for 30 min at room temperature. The proteins were analyzed by 7.5% SDS–PAGE and western blotting, using an anti-GFP antibody (Clontech). TIRF microscopy TIRF images were acquired using a TIRF illumination system (IX2-RFAEVA-2, Olympus) mounted on an inverted microscope equipped with an autofocus system (IX81-ZDC2; Olympus). A diode-pumped solid-state 488-nm laser (kyma488, 10 mW; Melles Griot) was used for total fluorescence illumination, and a 510-nm long-pass filter was used as an emission filter. Images were captured with a high-sensitivity EM-CCD camera (ImagEM; Hamamatsu Photonics) operated with the MetaMorph software (Molecular Devices). HEK293 cells expressing GFP-tagged TRPV4 constructs were plated onto poly- L -lysine-coated glass coverslips (Iwaki), and placed in a custom-designed chamber with HEPES-buffered saline (HBS) solution at room temperature. Co-immunoprecipitation assay At 30 h after transfection, HEK293 cells were lysed in RIPA buffer. The cell lysate was immunoprecipitated with the M2 monoclonal antibody to Flag (Sigma) in the presence of Protein A Sepharose beads (GE Healthcare) with rocking for 4 h at 4 °C. The immune complexes were washed three times with RIPA buffer and resuspended in SDS sample buffer containing 50 mM DTT, for 30 min at room temperature. The proteins were analyzed by 7.5% SDS–PAGE and western blotting using an anti-GFP antibody (Clontech). Measurement of [Ca 2+ ] i changes Fura-2 fluorescence was measured in HBS, containing 107 mM NaCl, 6 mM KCl, 1.2 mM MgSO 4 , 2 mM CaCl 2 , 11.5 mM glucose and 20 mM HEPES (pH adjusted to 7.4 with NaOH) [65] , [69] . Fluorescence images of the cells were recorded and analyzed with a video image analysis system (Aquacosmos; Hamamatsu Photonics), according to the manufacturer’s instructions. The ratio of 340:380 nm fluorescence was determined from the images, on a pixel-by-pixel basis. Fura-2 measurements were performed at 21±1 °C in HBS. The 340:380 ratios were converted to Ca 2+ concentrations by in vivo calibration using 5 μM ionomycin, as described previously [65] . Cell death assay The cells were incubated with 2 μg ml −1 propidium iodide (Sigma) in HBS solution. Fluorescence images of the cells were recorded and analyzed with a confocal laser-scanning microscope (FV500; Olympus), using the 488 nm line of an argon laser for excitation and either a 505–525-nm band-pass filter (GFP) or a 560-nm long-pass filter (propidium iodide) for emission. Statistical analyses All data are expressed as the mean±s.e.m. The data for each condition were obtained from at least three independent experiments. The statistical analyses were performed using the Student’s t -test. A value of P <0.05 was considered significant. Accession codes: Atomic coordinates and structure factors have been deposited in the Protein Data Bank ( http://www.pdb.org/ ) under accession codes 3W9F (IP 3 complex) and 3W9G (without IP 3 ). How to cite this article: Takahashi, N. et al. TRPV4 channel activity is modulated by direct interaction of the ankyrin domain to PI(4,5)P 2 . Nat. Commun. 5:4994 doi: 10.1038/ncomms5994 (2014).